Aneuploidy induces profound changes in gene expression, proliferation and tumorigenicity of human pluripotent stem cells Human pluripotent stem cells (hPSCs) tend to acquire genomic aberrations in culture, the most common of which is trisomy of chromosome 12. Here we dissect the cellular and molecular implications of this trisomy in hPSCs. Global gene expression analyses reveal that trisomy 12 profoundly affects the gene expression profile of hPSCs, inducing a transcriptional programme similar to that of germ cell tumours. Comparison of proliferation, differentiation and apoptosis between diploid and aneuploid hPSCs shows that trisomy 12 significantly increases the proliferation rate of hPSCs, mainly as a consequence of increased replication. Furthermore, trisomy 12 increases the tumorigenicity of hPSCs in vivo , inducing transcriptionally distinct teratomas from which pluripotent cells can be recovered. Last, a chemical screen of 89 anticancer drugs discovers that trisomy 12 raises the sensitivity of hPSCs to several replication inhibitors. Together, these findings demonstrate the extensive effect of trisomy 12 and highlight its perils for successful hPSC applications. Human pluripotent stem cells (hPSCs) are extraordinarily useful for basic biological research, and their unique characteristics render them promising for regenerative medicine [1] . During their culture propagation, however, both human embryonic stem cells (hESCs) and human induced pluripotent stem cells (hiPSCs) acquire genomic abnormalities that jeopardize their application for development and disease modelling, for drug screening and for cell therapies [2] , [3] , [4] . The genomic insults incurred to hPSCs in culture range in size from point mutations to full trisomies [2] , [3] , [4] . In fact, hESCs and hiPSCs tend to acquire typical large chromosomal aberrations, with the most prevalent one being the acquisition of an extra copy of chromosome 12 or of its short arm [5] , [6] , [7] , [8] , [9] , [10] . Trisomy 12-harbouring hPSCs (hereinafter referred to as T12-hPSCs) rapidly outcompete their normal counterparts in culture [5] , [6] , [7] , suggesting that this trisomy confers a strong selection advantage. Importantly, however, this selection advantage is cell type-specific, as trisomy 12 often arises in hPSCs but not in other types of stem cells [8] . A major concern regarding the potential impact of trisomy 12 on hPSCs is that it might increase their tumorigenic potential [4] , [11] . Of special concern is the fact that trisomy 12 is also the most common chromosomal aberration in various germ cell tumours (GCTs), which arise from cells that share some of their unique characteristics with hPSCs and are thus regarded as their in vivo cognates [12] . Extra copies of the short arm of chromosome 12 or of the entire chromosome were observed in ~75% of malignant ovarian GCTs [13] and in ~90% of testicular GCTs [14] . Moreover, a gene expression comparison of hESCs and human embryonic carcinoma cells revealed that genes from chromosome 12 are greatly over-represented among those that are significantly more highly expressed in embryonic carcinoma cells [15] . Despite these concerns, the functional consequences of trisomy 12 have not been comprehensively evaluated to date. In this study, we perform a thorough analysis of the impact of trisomy 12 on hPSCs. We first analyse the gene expression patterns of diploid and T12-hPSCs, and compare them to various GCT cell lines. Strikingly, this comparison reveals that trisomy 12 drastically affects the global gene expression profiles of hPSCs, making them more transcriptionally similar to those of GCTs. Next, we study the in vitro effects of trisomy 12. We find that T12-hPSCs grow faster in culture, and that this fast growth can be largely attributed to increased replication of the aneuploid cells. We then test the effects of trisomy 12 on teratoma formation in vivo , revealing that T12-hPSCs can give rise to more aggressive teratomas, or teratocarcinomas [16] , from which pluripotent cells can be recovered. Last, we screen diploid and aneuploid hPSCs against a library of Food and Drug Administration (FDA)-approved anticancer drugs, and find that T12-hPSCs are more sensitive to several cytotoxic replication inhibitors, further demonstrating their increased proliferation and suggesting that this property may be a potential liability of these aberrant cells. Trisomy 12 renders a GCT-like gene expression pattern in hPSCs We first composed a database of gene expression microarray data from diploid and aneuploid hPSCs, as well as GCT cell lines. The gene expression patterns of hPSCs were analysed by virtual karyotyping [17] , ensuring that the diploid hPSCs did not harbour any large chromosomal aberration, and that the aneuploid hPSCs harboured trisomy 12 as their sole large aberration. To prevent potential batch effects, each study contributed to the database either diploid or aneuploid samples, but not both. In total, we examined 24 diploid hPSC samples of 4 hESC and 6 hiPSC lines, from 11 different studies; 14 T12-hPSC samples of 3 hESC and 2 hiPSC lines, from 6 different studies (including new microarray data generated by us for the current study) and 21 GCT samples of 7 GCT cell lines, from 4 different studies. Three samples of a normal testis cell line were used as an outlier control. 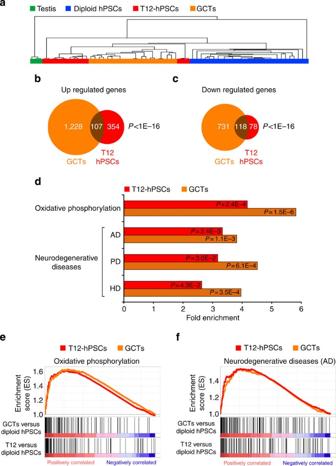Figure 1: Trisomy 12 renders global gene expression of hPSCs more similar to that of germ cell tumours (GCTs). (a) Unsupervised hierarchical clustering of diploid hPSCs, T12-hPSCs and various GCTs, based on the gene expression signature of all autosomal genes. (b) A Venn diagram presenting the genes that are upregulated in GCTs compared with diploid hPSCs and the genes that are upregulated in T12-hPSCs compared with diploid hPSCs. Significance of overlap is indicated (P<10−16, Pearson’sχ2goodness-of-fit test). (c) A Venn diagram presenting the genes that are downregulated in GCTs compared with diploid hPSCs and the genes that are downregulated in T12-hPSCs compared with diploid hPSCs. Significance of overlap is indicated (P<10−16, Pearson’sχ2goodness-of-fit test). (d) Perturbed biological pathways identified in GCTs and in T12-hPSCs, based on DAVID functional annotation enrichment analysis of the 500 most differentially expressed genes between GCTs and diploid hPSCs (orange) or between T12-hPSCs and diploid hPSCs (red).P-values are presented inside the bars. (e) GSEA enrichment plots for the Oxidative Phosphorylation KEGG pathway, by comparison of all autosomal genes between GCTs and diploid hPSCs (orange; NES=1.60,P=0.02), and between T12-hPSCs and diploid hPSCs (red; NES=1.58,P=0.03). (f) GSEA enrichment plots for the Alzheimer’s disease (AD) KEGG pathway, by comparison of all autosomal genes between GCTs and diploid hPSCs (orange; NES=1.59,P=0.02), and between T12-hPSCs and diploid hPSCs (red; NES=1.62,P=0.02). PD, Parkinson’s disease; HD, Huntington’s disease. Details about the analysed samples are provided in Supplementary Table 1 and Supplementary Fig. 1a . We subjected the global gene expression profiles to unsupervised hierarchical clustering, based on all of the autosomal probe sets. Strikingly, not only did T12-hPSCs cluster separately from diploid hPSCs, but they also clustered together with GCTs, indicating that their global gene expression profiles had become closer to those of GCT cell lines than to those of diploid hPSCs ( Fig. 1a ). Importantly, the global gene expression similarity between T12-hPSCs and GCT cell lines cannot be attributed to identical genome composition, as most (and probably all) of the GCT cell lines exhibit a complex karyotype, with multiple chromosomal gains and deletions ( Supplementary Table 1 ). However, as all GCTs overexpress genes from the short arm of chromosome 12 ( Supplementary Fig. 1b ), the presence of this gain in both T12-hPSCs and GCTs seems to explain the observed clustering to a large extent. Notably, although T12-hPSCs generally tend to be found at higher passages than diploid hPSCs, the altered gene expression signature is not a mere consequence of prolonged culture adaptation; high-passage diploid hPSCs clustered together with the other diploid hPSCs, whereas low-passage T12-hPSCs—including one hESC line with congenital trisomy 12 (ref. 18 )—clustered together with the other T12-hPSCs ( Fig. 1a and Supplementary Table 1 ). Figure 1: Trisomy 12 renders global gene expression of hPSCs more similar to that of germ cell tumours (GCTs). ( a ) Unsupervised hierarchical clustering of diploid hPSCs, T12-hPSCs and various GCTs, based on the gene expression signature of all autosomal genes. ( b ) A Venn diagram presenting the genes that are upregulated in GCTs compared with diploid hPSCs and the genes that are upregulated in T12-hPSCs compared with diploid hPSCs. Significance of overlap is indicated ( P <10 −16 , Pearson’s χ 2 goodness-of-fit test). ( c ) A Venn diagram presenting the genes that are downregulated in GCTs compared with diploid hPSCs and the genes that are downregulated in T12-hPSCs compared with diploid hPSCs. Significance of overlap is indicated ( P <10 −16 , Pearson’s χ 2 goodness-of-fit test). ( d ) Perturbed biological pathways identified in GCTs and in T12-hPSCs, based on DAVID functional annotation enrichment analysis of the 500 most differentially expressed genes between GCTs and diploid hPSCs (orange) or between T12-hPSCs and diploid hPSCs (red). P -values are presented inside the bars. ( e ) GSEA enrichment plots for the Oxidative Phosphorylation KEGG pathway, by comparison of all autosomal genes between GCTs and diploid hPSCs (orange; NES=1.60, P =0.02), and between T12-hPSCs and diploid hPSCs (red; NES=1.58, P =0.03). ( f ) GSEA enrichment plots for the Alzheimer’s disease (AD) KEGG pathway, by comparison of all autosomal genes between GCTs and diploid hPSCs (orange; NES=1.59, P =0.02), and between T12-hPSCs and diploid hPSCs (red; NES=1.62, P =0.02). PD, Parkinson’s disease; HD, Huntington’s disease. Full size image To examine whether the highly similar gene expression signatures of T12-hPSCs and GCT cell lines result from overexpression of genes that reside on chromosome 12, or from a wider influence that this trisomy might have on expression from other chromosomes, we repeated the unsupervised hierarchical clustering analysis without the chromosome 12 genes. Interestingly, excluding these genes had almost no effect on the results of these analyses ( Supplementary Fig. 1c ), indicating that trisomy 12 induces genome-wide gene expression alterations that render the global transcriptional programme of T12-hPSCs more similar to that of GCTs. To examine whether T12-hPSCs are more similar to GCTs than to other types of cancer, we compared the global expression signatures to those of two other types of cancer: ovarian adenocarcinoma (OA) [19] , which arises in the same tissue but is not a GCT, and chronic lymphocytic leukemia (CLL) [20] , a type of cancer in which trisomy 12 is also common [21] . A principal component analysis showed that T12-hPSCs and GCT cell lines cluster together, apart from the OA cell lines ( Supplementary Fig. 1d ), showing that T12-hPSCs are more similar to GCTs than to other cancer types. Moreover, the T12-CLL samples also clustered separately ( Supplementary Fig. 1d ), demonstrating that trisomy 12 alone is not sufficient to confer similar expression patterns in unrelated tumour types. Perturbation of common biological pathways in T12-hPSCs and GCTs We performed one-way analysis of variance (ANOVA) to obtain lists of differentially expressed genes between diploid hPSCs and either T12-hPSCs or GCTs. Using an expression fold change >2 and an false discovery rate (FDR)-corrected P -value <0.05, 461 probe sets were upregulated in T12-hPSCs compared with diploid hPSCs and 1,335 probe sets were upregulated in GCTs compared with diploid hPSCs; 107 of these probe sets were upregulated by both comparisons ( Fig. 1b , P <10 −16 , Pearson’s χ 2 goodness-of-fit test). Using the same thresholds, 196 probe sets were downregulated in T12-hPSCs compared with diploid hPSCs and 849 probe sets were downregulated in GCTs compared with diploid hPSCs; 118 of these probe sets were downregulated by both comparisons ( Fig. 1c , P <10 −16 , Pearson’s χ 2 goodness-of-fit test). We then subjected the 500 most differentially expressed probe sets between diploid hPSCs and T12-hPSC, as well as the 500 most differentially expressed probe sets between diploid hPSCs and GCTs, to DAVID functional annotation enrichment analyses. Remarkably, the same Kyoto Encyclopedia of Genes and Genomes (KEGG) pathways turned up in both analyses, indicating that CGTs and T12-hPSCs share perturbed biological pathways, which are related to energetic metabolism and to neural diseases ( Fig. 1d ). Gene set enrichment analysis (GSEA) with all expressed genes confirmed the enrichment for these KEGG pathways ( Fig. 1e,f ). Importantly, these pathways were not similarly perturbed in other tumours of the same tissue (OA) or in other tumours with trisomy 12 (T12-CLL). Last, we performed a PRomoter Integration in Microarray Analysis (PRIMA) analysis to identify transcription factors whose binding sites are enriched in both lists of differentially expressed genes. However, no enrichment was identified for any such transcription factor. Overexpression of Nanog was recently reported to result in impaired differentiation of mouse ESCs [22] . As NANOG resides inside the minimal recurrently gained region of human chromosome 12, and is significantly overexpressed in T12-hPSCs [7] , we next examined the potential role of NANOG in inducing the gene expression changes observed in T12-hPSCs. A comparison of the global gene expression changes of NANOG overexpressing cells (NANOG-OE hESCs) [23] to diploid hESCs revealed that the same biological pathways perturbed in T12-hPSCs, that is, oxidative phosphorylation and neural diseases, are also altered in NANOG-OE hESCs ( Supplementary Fig. 1e ), suggesting that NANOG overexpression is at least partly responsible for the gene expression perturbations observed in T12-hPSCs. Moreover, the list of 500 most differentially expressed probe sets in NANOG-OE hESCs significantly overlaps the list of 500 most differentially expressed probe sets in T12-hPSCs ( Supplementary Table 5 , P <10 −16 , Pearson’s χ 2 goodness-of-fit test). Nonetheless, most of the differentially expressed genes in T12-hPSCs are not differentially expressed in NANOG-OE hESCs, suggesting that trisomy 12 leads to a wider global gene expression change than NANOG overexpression alone. Trisomy 12 increases the proliferation of hPSCs We set out to determine the cellular consequences of trisomy 12. 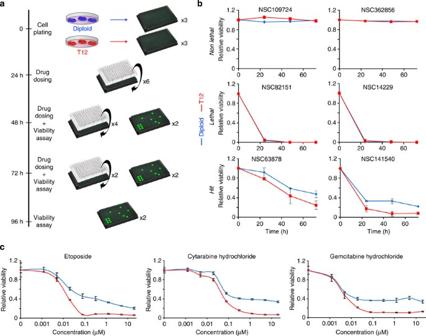Figure 5: Increased sensitivity of T12-hPSCs to DNA replication inhibitors revealed by screening 89 anticancer drugs. (a) A schematic representation of the drug screen performed with the FDA-approved Oncology Drugs Set II compound library against diploid and T12-hPSCs. (b) Relative cell number of diploid hPSCs (blue) or T12-hPSCs (red) exposed to drugs for 24, 48 or 72 h. Results are shown for two representative drugs of each category: ‘Non-lethal’, ‘Lethal’ and ‘Hit’ compounds. Drugs are mentioned by their NCI numeric identifiers (NSC numbers). Data represent an average of four replicates. (c) Relative cell number of diploid hPSCs (CSES10) and T12-hPSCs (CSES22) following a 48-h exposure to increasing concentrations of the three replication inhibitors that came up as ‘Hits’: etoposide, cytarabine hydrochloride and gemcitabine hydrochloride. Data represent an average of three replicates. Error bars represent standard errors. As trisomy 12 quickly takes over the culture [7] , and as T12-hPSCs often exhibit additional chromosomal aberrations [6] , [7] , [9] , it is challenging to capture the same cell line both in the diploid state and with trisomy 12 as its sole aberration. We therefore used two pairs of diploid and T12-hESCs for in vitro experiments: CSES10 versus CSES22 (refs 18 , 24 ) and HUES9 versus HUES7 (ref. 25 ). Each of these cell line pairs was derived and cultured in the same laboratory using the same culture conditions. We validated that CSES10 and HUES9 exhibit normal karyotypes, whereas CSES22 and HUES7 harbour trisomy 12 ( Fig. 2a ); HUES7 also harboured trisomy 17, which is commonly present in T12-hPSCs [5] , [6] , [7] ( Fig. 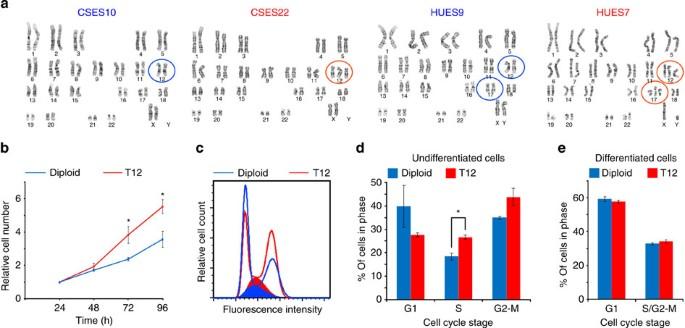2a ). Figure 2: Trisomy 12 increases the proliferation of hPSCs. (a) Karyotype analysis of the two pairs of diploid/aneuploid cell lines used for thein vitrocomparisons. Chromosomal aberrations are encircled. (b) Proliferation curves of diploid hPSCs (blue) and T12-hPSCs (red) in culture 24, 48, 72 and 96 h after plating. Data represent an average from four diploid hPSC lines (HUES1, HUES9, CSES10 and CSES7) and two T12-hPSC lines (HUES7 and CSES22). Each cell line was tested in triplicates. *P=0.018 at 72 h,P=0.036 at 96 h. (c) Cell cycle profiles of diploid hPSCs (blue) and T12-hPSCs (red) cultured under normal culture conditions, as evaluated by FACS. The highlighted areas represent the proportion of cells in S-phase. (d) Quantification of the proportion of cells in each of the cell cycle phases in diploid hPSCs (blue) and in T12-hPSCs (red). *P=0.019. Data represent an average of four independent experiments performed with the two pairs of diploid/aneuploid cell lines. (e) Quantification of the proportion of cells in the cell cycle phases in differentiating neurons from diploid hPSCs (blue) and from T12-hPSCs (red). Data represent an average of two independent experiments performed with the two pairs of diploid/aneuploid cell lines. Error bars represent standard errors.P-values obtained by one-tailed Student’st-test. Figure 2: Trisomy 12 increases the proliferation of hPSCs. ( a ) Karyotype analysis of the two pairs of diploid/aneuploid cell lines used for the in vitro comparisons. Chromosomal aberrations are encircled. ( b ) Proliferation curves of diploid hPSCs (blue) and T12-hPSCs (red) in culture 24, 48, 72 and 96 h after plating. Data represent an average from four diploid hPSC lines (HUES1, HUES9, CSES10 and CSES7) and two T12-hPSC lines (HUES7 and CSES22). Each cell line was tested in triplicates. * P =0.018 at 72 h, P =0.036 at 96 h. ( c ) Cell cycle profiles of diploid hPSCs (blue) and T12-hPSCs (red) cultured under normal culture conditions, as evaluated by FACS. The highlighted areas represent the proportion of cells in S-phase. ( d ) Quantification of the proportion of cells in each of the cell cycle phases in diploid hPSCs (blue) and in T12-hPSCs (red). * P =0.019. Data represent an average of four independent experiments performed with the two pairs of diploid/aneuploid cell lines. ( e ) Quantification of the proportion of cells in the cell cycle phases in differentiating neurons from diploid hPSCs (blue) and from T12-hPSCs (red). Data represent an average of two independent experiments performed with the two pairs of diploid/aneuploid cell lines. Error bars represent standard errors. P -values obtained by one-tailed Student’s t -test. Full size image The high prevalence of trisomy 12 in hPSC cultures, and its propensity to spread in culture within few passages, suggest that it must confer a selection advantage to the cells that harbour it, enabling them to rapidly outcompete diploid cells. We thus examined the proliferation rate of the diploid and aneuploid cells. Both of the T12-hPSC lines proliferated faster than their diploid counterparts, under normal culture conditions ( Fig. 2b ). These data indicate that trisomy 12 indeed confers a proliferative advantage to hPSCs. Such advantage can result from one or more of the following cellular mechanisms: increased replication, decreased cell death and/or reduced differentiation in culture. To examine which of these mechanisms underlies the observed growth advantage of T12-hPSCs, we used flow cytometry to analyse the cell cycle, the spontaneous apoptosis rate and the spontaneous differentiation rate of diploid (CSES10 and HUES9) and aneuploid (CSES22 and HUES7) cells. Measuring the expression of the pluripotency marker TRA-1–60 exposed a somewhat reduced tendency of T12-hPSCs towards spontaneous differentiation ( Supplementary Fig. 2a ). An apoptosis assay also revealed a slightly decreased apoptosis rate in T12-hPSCs ( Supplementary Fig. 2b ). Most strikingly, however, cell cycle analysis unraveled a significant change in the cell cycle profile of T12-hPSCs: the proportion of cells at S-phase was significantly higher in both T12-hPSC lines, compared with their diploid counterparts ( Fig. 2c,d ; P =0.019, one-tailed Fisher’s exact test). We therefore conclude that trisomy 12 confers proliferation advantage to T12-hPSCs mainly through increasing their replication in culture. Interestingly, after 10 days of neural differentiation the proportion of replicating cells was similar between neural cells derived from diploid and from T12-hPSCs ( Fig. 2e ), suggesting that the proliferation advantage conferred by trisomy 12 may be restricted to the undifferentiated state. A comparison of the cell cycle profiles between diploid and NANOG-OE hESCs revealed very similar cell cycle profiles ( Supplementary Fig. 2c ), suggesting that overexpression of NANOG alone is not sufficient to confer the significant proliferation advantage observed in T12-hPSCs, at least under normal culture conditions. Teratomas from T12-hPSCs share a distinct gene expression profile Next, we examined the tumorigenicity of T12-hPSCs in vivo , using teratoma formation assays. Diploid and aneuploid hPSCs were injected under the kidney capsule of immunodeficient mice, and tumours were obtained 3–4 weeks later. In total, we generated nine teratomas from six diploid undifferentiated hESCs (CSES2, CSES4, CSES7, CSES12, CSES15, CSES25, CSES26), three teratomas from one hESC line with congenital trisomy 12 (CSES45, ref 18 ) and one teratoma from one hESC line with acquired trisomy 12 (CSES22). We also generated four teratomas from early passage diploid hiPSCs (hiPSC18, ref. 26 ) and four teratomas from late passage T12-hiPSCs of the same cell line [7] . A detailed list of teratomas appears in Supplementary Table 2 . RNA was derived from multiple teratomas and subjected to Affymetrix U133Plus2 gene expression microarrays. In total, we compared gene expression microarrays from five representative diploid hPSC-derived teratomas to those from three representative T12-hPSC-derived teratomas ( Supplementary Table 2 ). Gene expression-based moving average plot suggested that T12-hPSC teratomas present a distinct gene expression signature throughout the entire autosomal genome ( Fig. 3a ). As a similar moving average plot of undifferentiated hPSCs did not exhibit such a marked difference between the diploid and aneuploid cells ( Supplementary Fig. 1f ), these data suggest that teratomas from T12-hPSCs become more distinct from their diploid counterparts throughout their differentiation. Unsupervised hierarchical clustering, based on all of the autosomal probe sets, indeed divided the teratomas into two main clusters according to their trisomy 12 status ( Fig. 3b ). Of special interest is the fact that the teratoma from CSES45, a cell line with congenital trisomy 12, clustered together with the rest of the T12-hPSC teratomas ( Fig. 3b ), indicating that it is really the existence of an extra copy of chromosome 12 (rather than other potential effects of culture adaptation) that underlies the unique gene expression signature of these teratomas. Moreover, virtual karyotyping analysis revealed that the teratoma from CSES26 had acquired trisomy of chromosome 20; this teratoma, however, clustered together with the diploid teratomas ( Fig. 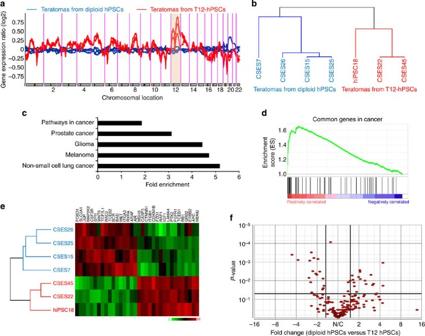3a,b ), suggesting that the identified gene expression signature is not shared by any teratoma from aneuploid hPSCs, but is unique to those from T12-hPSCs. Figure 3: Teratomas from T12-hPSCs share a distinct gene expression profile and differentially express cancer-related genes. (a) Gene expression-based moving average plot of teratomas from diploid hPSCs (blue) and from T12-hPSCs (red). (b) Unsupervised hierarchical clustering of teratomas from diploid and T12-hPSCs, based on the gene expression signature of all autosomal genes. (c) Perturbed biological pathways identified in teratomas from T12-hPSCs, based on DAVID functional annotation enrichment analysis of the 500 most differentially expressed genes. (d) GSEA enrichment plot for the ‘common genes in cancer’ gene set, enriched in T12-hPSCs. (e) Unsupervised hierarchical clustering of teratomas from diploid hPSCs and T12-hPSCs, based on the genes that belong to the ‘pathways in cancer’ KEGG biological pathway. The heat map presents the subset of genes in this pathway that are differentially expressed between diploid and T12-hPSC-derived teratomas. (f) Volcano plot of the genes that belong to the ‘pathways in cancer’ KEGG biological pathway. 34 (17%) of these genes are differentially expressed between diploid and T12-hPSC-derived teratomas (fold change >2,P<0.05, Pearson’sχ2goodness-of-fit test). Figure 3: Teratomas from T12-hPSCs share a distinct gene expression profile and differentially express cancer-related genes. ( a ) Gene expression-based moving average plot of teratomas from diploid hPSCs (blue) and from T12-hPSCs (red). ( b ) Unsupervised hierarchical clustering of teratomas from diploid and T12-hPSCs, based on the gene expression signature of all autosomal genes. ( c ) Perturbed biological pathways identified in teratomas from T12-hPSCs, based on DAVID functional annotation enrichment analysis of the 500 most differentially expressed genes. ( d ) GSEA enrichment plot for the ‘common genes in cancer’ gene set, enriched in T12-hPSCs. ( e ) Unsupervised hierarchical clustering of teratomas from diploid hPSCs and T12-hPSCs, based on the genes that belong to the ‘pathways in cancer’ KEGG biological pathway. The heat map presents the subset of genes in this pathway that are differentially expressed between diploid and T12-hPSC-derived teratomas. ( f ) Volcano plot of the genes that belong to the ‘pathways in cancer’ KEGG biological pathway. 34 (17%) of these genes are differentially expressed between diploid and T12-hPSC-derived teratomas (fold change >2, P <0.05, Pearson’s χ 2 goodness-of-fit test). Full size image As in the analysis of undifferentiated hPSCs discussed above, we examined whether the T12-hPSC teratoma gene expression signatures result from overexpression of genes that reside on chromosome 12 only, or from a wider transcriptional shift. We therefore repeated the unsupervised hierarchical clustering analysis without the chromosome 12 genes. Here again, excluding these genes had very little effect on the results of these analyses ( Supplementary Fig. 3a ), indicating that trisomy 12 induces genome-wide gene expression alterations in the derived teratomas. We performed one-way ANOVA to obtain a list of differentially expressed genes between teratomas from diploid and aneuploid hPSCs. Using an expression fold change >2 and an FDR-corrected P -value <0.05, 1,198 probe sets were upregulated and 397 probe sets were downregulated in T12-hPSC teratomas. The 500 most upregulated probe sets in T12-hPSC teratomas were subjected to DAVID functional annotation enrichment analysis. Interestingly, enrichment was revealed for several cancer-related KEGG pathways ( Fig. 3c ). Moreover, GSEA with all expressed genes identified the ‘Common genes in cancer’ gene set as the most significantly enriched gene set in T12-hPSC teratomas (normalized enrichment score=1.92, P <10 −4 by GSEA statistical analysis; Fig. 3d ). We therefore decided to closely examine the gene list of the ‘Pathways in human cancer’ KEGG pathway [27] . A total of 200 of these 240 genes are also included in the HG_U133Plus2 microarray platform. Unsupervised hierarchical clustering based on these probe sets correctly separated between diploid and T12-hPSC-derived teratomas ( Fig. 3e ), and 34 (17%) of these genes were differentially expressed between these teratomas (fold change >2, P <0.05, Pearson’s χ 2 goodness-of-fit test; Fig. 3e,f and Supplementary Table 3 ). Together, these data reveal an increased expression of cancer-related genes in teratomas from T12-hPSCs. Pluripotent stem cells can be recovered from T12-hPSC teratomas We next hypothesized that T12-hPSC-derived teratomas might contain foci of undifferentiated pluripotent cells, which are normally not present in diploid hPSC-derived teratomas and that would further increase their tumorigenicity. Teratomas generated from diploid and T12-hPSCs were dissected and analysed by immunohistochemistry with an antibody against the pluripotency marker OCT-4. Whereas no significant expression of OCT-4 could be detected in the diploid hPSC-derived teratomas, several of the T12-hPSC-derived teratomas, and especially the teratomas from the high-passage T12-hiPSC line hiPS18, contained residual undifferentiated cells ( Fig. 4a ). Immunostaining for two additional pluripotency markers, NANOG and SOX-2, confirmed the existence of undifferentiated cells in T12-hPSC-derived teratomas ( Supplementary Fig. 3b ). Undifferentiated cells were similarly identified in tumours from the GCT cell line TERA1 ( Supplementary Fig. 3c ). These results were corroborated by quantitative reverse transcription–PCR, which revealed higher expression of OCT-4 and NANOG in some of the T12-hPSC-derived teratomas ( Fig. 4b and Supplementary Fig. 3d ). In line with the existence of undifferentiated cells in T12-hPSCs, teratomas from high-passage T12-hiPS18 cells grew faster than their diploid counterparts, reaching a larger size at the same time point ( Fig. 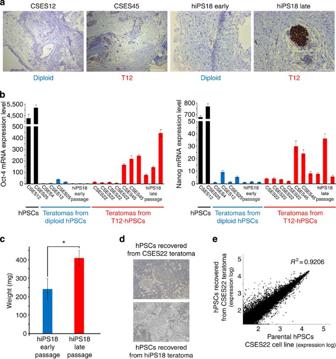4c ). Figure 4: Pluripotent stem cells can be recovered from T12-hPSC teratomas. (a) Histological sections of teratomas from diploid hPSCs (CSES12 and hiPS18 from an early passage) and T12-hPSCs (CSES45 and hiPS18 from a late passage), stained with an antibody against the pluripotency marker OCT-4. Scale bar, 100 μm for CSES12 and CSES45, 50 μm for hiPS18. (b) Quantification by reverse transcription–PCR ofOCT-4andNANOGmRNA expression levels in undifferentiated hPSCs, teratomas from diploid hPSCs and teratomas from T12-hPSCs. Error bars represent standard errors. (c) Weight comparison of teratomas from diploid hPSCs (hiPS18 from an early passage) and T12-hPSCs (hiPS18 from a late passage), obtained at the same time point (4 weeks following cell injection). *P=0.033, one-tailed Student’st-test. Data represent an average of four teratomas of each cell type. (d) Microscopy images of pluripotent-like cells recovered from T12-hPSC-derived teratomas. Scale bar, 100 μm. (e) Gene expression-based scatter-plot analysis of pluripotent cells recovered from T12-hPSC-derived teratomas versus their parental undifferentiated cells line (CSES22). Figure 4: Pluripotent stem cells can be recovered from T12-hPSC teratomas. ( a ) Histological sections of teratomas from diploid hPSCs (CSES12 and hiPS18 from an early passage) and T12-hPSCs (CSES45 and hiPS18 from a late passage), stained with an antibody against the pluripotency marker OCT-4. Scale bar, 100 μm for CSES12 and CSES45, 50 μm for hiPS18. ( b ) Quantification by reverse transcription–PCR of OCT-4 and NANOG mRNA expression levels in undifferentiated hPSCs, teratomas from diploid hPSCs and teratomas from T12-hPSCs. Error bars represent standard errors. ( c ) Weight comparison of teratomas from diploid hPSCs (hiPS18 from an early passage) and T12-hPSCs (hiPS18 from a late passage), obtained at the same time point (4 weeks following cell injection). * P =0.033, one-tailed Student’s t -test. Data represent an average of four teratomas of each cell type. ( d ) Microscopy images of pluripotent-like cells recovered from T12-hPSC-derived teratomas. Scale bar, 100 μm. ( e ) Gene expression-based scatter-plot analysis of pluripotent cells recovered from T12-hPSC-derived teratomas versus their parental undifferentiated cells line (CSES22). Full size image We next tested whether undifferentiated pluripotent cells could be recovered from T12-hPSC teratomas. Teratomas were explanted, and cells were grown in vitro under normal hPSC culture conditions. Remarkably, pluripotent-like cells soon appeared in the teratoma cell cultures from T12-hiPSC cell lines CSES22 and hiPS18 ( Fig. 4d ). We therefore compared the ability to recover undifferentiated cells between diploid and aneuploid teratomas. Recovery attempts were made with an average of three teratomas of each cell line. Pluripotent-like cells could be recovered from 4 out of 17 (23.5%) teratomas corresponding to only 1 out of 5 (20%) diploid hPSC lines; in contrast, pluripotent-like cells could be recovered from 7 out of 10 (70%) teratomas representing all 3 of 3 (100%) T12-hPSC lines ( Supplementary Fig. 4a ). This difference is statistically significant ( P =0.024, one-tailed Fisher’s exact test). It may well be that the single diploid cell line whose teratomas gave rise to pluripotent-like cells had acquired chromosomal aberrations (or other genetic or epigenetic abnormalities) during its in vivo differentiation. RNA from the T12-teratoma-derived cell lines was subjected to gene expression microarrays. Gene expression-based scatter plots showed that some recovered cell lines were highly similar to their parental hPSC line ( Fig. 4e ) and expressed hallmark pluripotency markers ( Supplementary Fig. 4b ), whereas others were only partially similar to their parental cell line and did not regain high expression of all pluripotency markers ( Supplementary Fig. 4c,d ). Together, these data indicate that T12-hPSCs can lead to the formation of distinct, potentially more aggressive tumours, from which fully or partially undifferentiated cells can be recovered. Increased sensitivity of T12-hPSCs to DNA replication inhibitors Considering the global gene expression signature of T12-hPSCs, and their increased proliferation and tumorigenicity, we reasoned that T12-hPSCs might be more sensitive to some anticancer drugs, compared with their diploid counterparts. Distinct drug response could potentially shed light on differentially regulated pathways between diploid and aneuploid hPSCs. Furthermore, selective growth inhibition or elimination of aberrant hPSCs could be valuable for the routine propagation of hPSCs in culture. We therefore decided to examine the response of diploid and aneuploid hPSCs to anticancer drugs. We started by examining three compounds that were recently shown to inhibit aneuploid cells: the energy stress-inducing agent AICAR (aminoimidazole carboxamide ribonucleotide), the protein folding inhibitor 17-AAG (17-(Allylamino)-17-demethoxygeldanamycin) and the autophagy inhibitor chloroquine [28] . These compounds were shown to induce apoptosis in aneuploid mouse embryonic fibroblasts (MEFs), and the former two also inhibited aneuploid human cancer cells [28] . Cell viability measurements following a 24-h exposure of diploid and T12-hPSCs to these compounds (at the same concentrations found to be effective against aneuploid cancer cells) showed no differential response ( Supplementary Fig. 5a ). These findings are in line with a previous work that reported that hESCs with trisomy 21 did not respond differently to these drugs [29] . Next, we went on to screen the FDA-approved Oncology Drugs Set II compound library (Developmental Therapeutics Program, NCI, USA). This library contains 89 small molecules approved by the FDA for various cancer indications. Diploid or aberrant hPSCs were plated in 96-well culture plates without feeder cells (using mTeSR1 culture medium), and exposed to the drugs at a high concentration (20 μM) for 24, 48 or 72 h (see Methods). The number of viable cells in each well was measured at each time point using an ATP-based cell viability assay (CellTiter-Glo). As a positive control, three wells in each plate were exposed to the cytotoxic drug amsacrine hydrochloride that had been previously shown to eliminate undifferentiated hPSCs [30] . As a negative control, three wells in each plate were exposed to dimethylsulphoxide (DMSO; 1%). For each drug, the viability of the exposed cells was normalized to the negative controls at each time point. Two pairs of diploid and T12-hPSCs (CSES10 versus CSES22 and HUES9 versus HUES7) were screened twice each. A schematic representation of the screen is presented in Fig. 5a . Figure 5: Increased sensitivity of T12-hPSCs to DNA replication inhibitors revealed by screening 89 anticancer drugs. ( a ) A schematic representation of the drug screen performed with the FDA-approved Oncology Drugs Set II compound library against diploid and T12-hPSCs. ( b ) Relative cell number of diploid hPSCs (blue) or T12-hPSCs (red) exposed to drugs for 24, 48 or 72 h. Results are shown for two representative drugs of each category: ‘Non-lethal’, ‘Lethal’ and ‘Hit’ compounds. Drugs are mentioned by their NCI numeric identifiers (NSC numbers). Data represent an average of four replicates. ( c ) Relative cell number of diploid hPSCs (CSES10) and T12-hPSCs (CSES22) following a 48-h exposure to increasing concentrations of the three replication inhibitors that came up as ‘Hits’: etoposide, cytarabine hydrochloride and gemcitabine hydrochloride. Data represent an average of three replicates. Error bars represent standard errors. Full size image After validating the high quality of the screen ( Z ′ values ranging from 0.82 to 0.88), the effect of each drug was compared between diploid and T12-hPSCs, and the compounds were divided into three groups: ‘Non-lethal’ compounds: drugs that did not inhibit the growth of hPSCs at any time point; ‘Lethal’ compounds: drugs that were highly and equally cytotoxic towards all hPSCs; ‘Hit’ compounds: drugs with stronger inhibitory effect towards the aberrant T12-hPSCs. Drugs that did not meet the stringent criteria to get included in any of these groups, and those that showed inconsistent effects, were excluded from further analysis (see Methods). In total, out of 89 drugs, 20 came up as ‘lethal’, 13 as ‘non-lethal’ and 5 as ‘hits’ ( Supplementary Table 4 ). Representative graphs for each category are presented in Fig. 5b . Of note, as the screen was performed at one concentration, we cannot rule out that some of the ‘non-lethal’ or ‘lethal’ compounds would exhibit a differential cytotoxicity at higher or lower concentrations, respectively. The ‘hit’ compounds, on the other hand, are likely to have an even stronger differential effect at optimal concentrations, and we thus decided to focus on their confirmation. Previously, the drugs included in the Approved Oncology Drug Set were divided into 5 mechanistic categories (replication inhibitors, DNA damaging agents, enzymatic inhibitors, hormones and growth inhibitors, miscellaneous) and 18 sub-categories [31] . We correlated our screen results with these functional categories ( Table 1 ). Interestingly, the three most differential compounds that came up as ‘hits’ in the screen belonged to the group of DNA replication inhibitors: etoposide, a DNA topoisomerase II poison; cytarabine hydrochloride, a nucleoside analogue; and gemcitabine hydrochloride, another nucleoside analogue. Although these drugs are also cytotoxic towards diploid hPSCs, they affect T12-hPSCs more significantly. We confirmed this differential effect by exposing diploid and T12-hPSCs to multiple concentrations of each of these drugs ( Fig. 5c and Supplementary Fig. 5b ). Thus, the differential response of T12-hPSCs to replication inhibitors is consistent with the increased replication that we observed in these cells. Table 1 Library screen results divided by drugs mechanism of action. Full size table Despite its prevalence in hPSC cultures, as well as in various GCTs, the cellular consequences of trisomy 12 have not been extensively studied in pluripotent cells. Although one study reported that teratomas from T12-hESCs are not significantly different in their gross composition [32] , another study reported that T12-hESCs undergo abnormal cell division [33] ; both studies, however, assessed only one cell line each, using limited experimental assays. In the current study, we compared the global gene expression signatures of dozens of hPSC and GCT cell lines, and revealed that trisomy 12 renders hPSCs more transcriptionally similar to GCTs. Surprisingly, this effect is not merely a consequence of overexpression of genes that reside on chromosome 12; rather, trisomy 12 induces a genome-wide expression change that shifts the transcriptional programme of T12-hPSCs away from that of their diploid counterparts and towards that of GCTs. Interestingly, the differentially expressed genes between diploid and T12-hPSCs, and between diploid hPSCs and GCTs, converge on the same biological pathways related to cell metabolism and to neural diseases. Recent studies have reported multiple metabolic pathways that are uniquely regulated in pluripotent cells [30] , [34] , [35] , and enrichment for metabolic genes was also found in a gene expression comparison between naïve and primed mouse ESCs [36] . It will thus be interesting to further compare the metabolism of diploid and T12-hPSCs, in order to identify specific metabolic alterations that might be important for the selection advantage conferred by this trisomy. The enrichment for pathways related to neural diseases highlights a potential danger in using T12-hPSCs for studying these diseases. Of note, overexpression of Nanog was recently reported to result in impaired differentiation of mouse ESCs [22] , and we found that NANOG overexpression leads to the perturbation of the same biological pathways perturbed in T12-hPSCs. Future studies are required to further characterize the differentiation capacity of T12-hPSCs towards the neural lineage, and to examine whether this effect is indeed regulated by NANOG . More broadly, several pluripotency genes (such as, NANOG and GDF3 ) and oncogenes (for example, KRAS ) have been suggested to underlie the selection advantage conferred by trisomy 12 (refs 5 , 6 , 7 ). Our findings should help to identify the combination of genes on chromosome 12 that drive the drastic gene expression changes and consequently mediate the cellular phenotypes observed in T12-hPSCs. Our in vitro studies revealed that T12-hPSCs proliferate faster than diploid hPSCs, which can account for the fact that these aberrant cells rapidly outcompete the normal cells in culture [6] , [7] . This proliferation advantage is mostly due to increased replication in T12-hPSCs. Although increased replication enables T12-hPSCs to take over the culture, it also makes them more vulnerable to replication inhibitors. An intriguing hypothesis, which awaits experimental validation, is that this vulnerability is mediated through increased replication stress in T12-hPSCs. It also remains to be seen whether the stronger response of T12-hPSCs to replication inhibitors can be harnessed to practical applications (that is, the prevention of trisomy 12 accumulation in culture); the selective inhibitors that we have identified are also cytotoxic towards diploid hPSCs, and they might jeopardize their genomic integrity, thus hindering their potential use in routine hPSC culture propagation. Last, our in vivo differentiation studies revealed that teratomas from T12-hPSCs differ from diploid teratomas in their global gene expression signature, as well as in the expression of cancer-related genes. Moreover, undifferentiated cells could be recovered from these aberrant T12-hPSC-derived tumours, suggesting that these tumours could be aptly described as teratocarcinomas [16] . These findings are consistent with the in vitro data, with the high prevalence of trisomy 12 in GCTs [8] , and with the GCT-like gene expression signature of T12-hPSCs. These results also resemble data obtained with teratomas from partially transformed hPSCs [37] . Collectively, our findings demonstrate that trisomy 12 increases the tumorigenicity of hPSCs, and highlight the caution that is warranted when working with such aberrant cells. As trisomy 12 is the most common chromosomal aberration in hPSCs, these findings call for tight monitoring of hPSC genomic integrity throughout their culture propagation, both for their proper use in basic research and for their safe application in regenerative medicine. Cell culture CSES [18] , [24] and HUES [25] hESCs and hiPS18 hiPSCs [26] were cultured under standard culture conditions, as previously described [7] . In short, cells were grown on mitomycin C-treated MEF feeder layer (obtained from 13.5-day embryos) in 85% KnockOut Dulbecco’s modified Eagle’s medium (Invitrogen) supplemented with 15% KnockOut SR (a serum-free formulation; Invitrogen), 1 mM glutamine, 0.1 mM β-mercaptoethanol (Sigma-Aldrich), 1% nonessential amino acids stock (Invitrogen), penicillin (50 U ml −1 ), streptomycin (50 μg ml −1 ) and FGF2 (Invitrogen). Cells were passaged using trypsin-EDTA (Sigma-Aldrich). Neural differentiation was induced by withdrawal of basic fibroblast growth factor and addition of retinoic acid (Sigma-Aldrich) to the medium at a final concentration of 1 μM. Karyotyping The night before the procedure, hESC culture medium was replaced. KaryoMAX colcemid (Invitrogen) was added directly to the plate of cells during the following morning (at final concentration of 100 ng ml −1 ), and cells were incubated for 30 min at 37 °C (with 5% CO 2 ). Cells were then trypsinized, treated with hypotonic solution and fixed. Metaphases were spread on microscope slides, and by using standard G banding technique, the chromosomes were classified according to the International System for Human Cytogenetic Nomenclature. RNA isolation, reverse transcription and quantitative real-time PCR Total RNA was extracted using RNeasy mini kit (Qiagen). Quantitative expression analysis was performed by RTqPCR on a Bio-Rad C1000 Thermal Cycler equipped with a CFX96 Real-Time System, with the iQ SYBR Green kit (Bio-Rad). Template cDNA was prepared from 2 μg of total RNA using the Maxima First Strand cDNA kit (Fermentas). GAPDH (glyceraldehyde 3-phosphate dehydrogenase) or ACTB (actin beta) were used as the endogenous control. Primer sequences for OCT-4: 5′-AGTGAGAGGCAACCTGGAGA-3′ (forward) and 5′-ACACTCGGACCACATCCTTC-3′ (reverse); for NANOG: 5′-GATTTGTGGGCCTGAAGAAA-3′ (forward) and 5′-CAGATCCATGGAGGAAGGAA-3′ (reverse); for GAPDH: 5′-CAATGACCCCTTCATTGACC-3′ (forward) and 5′-GACAAGCTTCCCGTTCTCAG-3′ (reverse); for ACTB: 5′-TCCCTGGAGAAGAGCTACGA-3′ (forward) and 5′-AGGAAGGAAGGCTGGAAGAG-3′ (reverse). Global gene expression analysis Total RNA was extracted from undifferentiated hPSCs, from hPSC-derived teratomas and from cell lines recovered from hPSC-derived teratomas, using RNeasy mini kit (Qiagen), according to the manufacturer’s protocol. RNA was subjected to Human Genome U133 Plus 2.0 microarray platform (Affymetrix); washing and scanning were performed according to the manufacturer’s protocol. Original microarray data are accessible at the NCBI Gene Expression Omnibus database under the accession number GSE51455 . In addition, microarray data of undifferentiated hPSCs from previous studies were downloaded from the Gene Expression Omnibus database (accession numbers are detailed in Supplementary Table 1 ). Each study contributed to the database either diploid or T12-hPSCs. Arrays were normalized using MAS5 algorithm in the Affymetrix Expression Console. Probe sets absent in both diploid and aberrant hPSCs were filtered out by the MAS5 Absent/Present call. Probe sets with expression values lower than 200 were raised to this level. The karyotype of the analysed cell lines was validated by virtual karyotyping [17] . Genome-wide moving average plots were obtained using the CGH-Explorer ( http://heim.ifi.uio.no/bioinf/Projects/ CGHExplorer). ANOVA and unsupervised hierarchical clustering analyses were performed using the Partek Genomics Suite version 6.3 (Partek). Following ANOVA, batch effect was removed using the PARTEK ‘batch effect removal’ procedure. These analyses were performed by using all expressed probe sets, by using the expressed probe sets that are not encoded from chromosome 12, or by using the expressed probe sets that are encoded from chromosome 12 only. Lists of differentially expressed genes between various conditions (diploid hPSCs versus T12-hPSCs, diploid hPSCs versus GCT cell lines, diploid hPSC-derived teratomas versus T12-hPSC-derived teratomas, parental undifferentiated T12-hPSCs versus recovered undifferentiated cells from teratomas) were derived by applying the following thresholds: fold-change >2, FDR-corrected P -value <0.05. To detect significantly over-represented KEGG pathways, the lists of differentially expressed genes were subjected to the DAVID functional annotation clustering tool ( http://david.abcc.ncifcrf.gov ). To detect significantly over-represented transcription binding sites, the lists of differentially expressed genes were subjected to PRIMA analysis ( http://acgt.cs.tau.ac.il/prima/ ). GSEA was performed using the GSEA software ( http://www.broadinstitute.org/gsea/index.jsp ). hESCs overexpressing NANOG [23] were used to compare the 500 most differentially expressed genes in T12-hPSCs to that in NANOG-EO-ESCs. Cell viability and proliferation assays Following trypsinization, cells were plated as single cells at a density of ~125 K cells per cm 2 . Relative cell numbers were determined by fixating the cells with 0.5% glutardialdehyde (Sigma-Aldrich) and staining with methylene blue (Sigma-Aldrich) dissolved in 0.1 M boric acid (pH 8.5). Colour extraction was performed using 0.1 M hydrochloric acid, and the staining (which is proportional to cell number) was quantified by measuring absorbance at 650 nm. 17-AAG, AICAR and chloroquine were purchased from Sigma-Aldrich. FACS analysis For pluripotency analysis, cells were incubated on ice with TRA-1-60-PE antibody (1:40, BD Biosciences), washed and data were acquired and analysed using FACSAria Cell-Sorting System (Becton Dickinson). For quantification of apoptosis, Annexin V-FITC Apoptosis Detection Kit (eBioscience) was used, according to the manufacturer’s instructions. Acquisition and analysis were performed using FACSAria Cell-Sorting System (Becton Dickinson). For cell cycle analysis, cells were trypsinized and incubated in methanol at −20 °C for 2 h. RNA digestion was performed with 200 μg ml −1 RNase A (Sigma-Aldrich) for half an hour at room temperature (RT). Cells were stained with 50 μg ml −1 propidium iodide (PI) for 10 min at 25 °C, and were taken for FACS analysis. Acquisition was performed using FACSAria Cell-Sorting System (Becton Dickinson), and analysis was performed with the FlowJo software ( http://www.flowjo.com/ ). Cell cycle analysis of the differentiated neural cells was performed using the FACSAria Cell-Sorting System (Becton Dickinson), using the size of the cells as means to separate undifferentiated from differentiating cells. Tumour formation and analysis Undifferentiated hPSCs were collected with trypsin (Sigma-Aldrich). ~3 × 10 6 cells were re-suspended in 50–100 μl of PBS and injected under the kidney capsule of 6- to 8-week-old nude mice. Three to four weeks after injection, mice were killed, the formation of tumours was examined and the resulting teratomas were photographed, dissected and divided into three portions: one for RNA, one for immunohistochemistry and one for culture. The portion reserved for isolation of RNA was immediately homogenized in RLT buffer (RNeasy Mini kit, Qiagen) using a Polytron PT 1,200 E system (Kinematica). The second portion to use for immunostaining was fixed overnight in 10% formalin, and mounted in paraffin. The remnant portion was collected in sterile DMEM, chopped manually with a scalpel blade and seeded on a monolayer of mitomycin-inactivated MEFs. When hESC-like colonies appeared, they were manually picked and transferred to a plate with a new MEF feeder layer. HESC-like cells were thus expanded manually for the first 2–3 passages, and were then passaged using collagenase IV (STEMCELL Technologies). GCT TERA1 cells were similarly harvested and injected subcutaneously into immunodeficient mice. Four weeks after injection, mice were killed, the formation of tumours was examined and the resulting tumours were photographed, dissected and stained. All experimental procedures in animals were in accordance with institutional guidelines as approved by the Cedars-Sinai Medical Center Institutional Animal Care and Use Committee, according to protocol #2,182. Immunohistochemistry Four-micron sections were permeabilized with 1% Triton X-100 for 1 h at RT, washed twice with PBS and incubated with blocking solution (0.1% Triton X-100+10% normal goat serum in PBS) for another hour at RT. Rabbit monoclonal anti-OCT-4 antibody (Cell Signaling; 1:100) was diluted in blocking solution and incubated overnight at 4 °C, followed by incubation with horseradish peroxidase-conjugated goat anti-rabbit IgG (Santa Cruz). Colour development was performed with DAB (3,3'-diaminobenzidine), and hematoxilin–eosin was used for histological staining of the tissue. For fluorescence immunohistochemistry, sections were fixed in formaldehyde (4%), stained with primary antibodies (rabbit anti-OCT-4 (Santa Cruz; 1:50); rabbit anti-NANOG (Santa Cruz; 1:50); goat anti-SOX-2 (Santa-Cruz; 1:50)), washed and stained with secondary antibodies (Jackson Immunoresearch laboratories; 1:100). Microscopy images were taken using an Olympus IX81 microscope (Olympus). Chemical drug library screening The Approved Oncology Drugs Set II was obtained from the NCI/DTP Open Chemical Repository Collection ( http://dtp.nci.nih.gov/repositories.html ), in a 96-well format. Positive and negative controls were added to three empty wells each, by adding 20 μl of 10 mM Amsacrine hydrochloride (Sigma-Aldrich) or 100% DMSO (Sigma-Aldrich), respectively. The compound plate was divided into eight 96-well Nunc plates (Thermo Scientific), containing 2.5 μl of each compound. At day 0, undifferentiated hPSCs (CSES10, CSES22, HUES9, HUES7) were harvested and seeded on six 96-well Nunc tissue culture plates pre-coated with Matrigel (BD Biosciences), at a density of 2.0 × 10 −5 cells per well. Cell numbers were adjusted by the relative cell growth at time of seeding. Cells were grown in a medium composed of standard ES culture medium [7] and mTeSR1 medium (STEMCELL Technologies) at a 1:1 ratio. At day 1 (+24 h), the compound plate was diluted in culture medium at a ratio of 1:110, medium in the assay plates was replaced, and diluted compounds were added to the assay plates at a final compound concentration of 20 μM (1% DMSO). At day 2 (+48 h), two plates were subjected to a cell viability assay, and medium in the remaining four plates was replaced with fresh compound-containing medium. At day 3 (+72 h), two plates were subjected to a cell viability assay, and medium in the remaining two plates was replaced with fresh compound-containing medium. At day 4 (+96 h), the remaining two plates were subjected to a cell viability assay. Cell viability was determined using CellTiter-Glo Luminescent Cell Viability Assay (Promega), according to the manufacturer’s protocol. Luminescence was quantitated using Envision Multilabel Plate Reader (Perkin Elmer). The assay plates were incubated at 37 °C, 5% CO 2 for the entire time of the screen, except from the time required for liquid handling. All liquid transfer steps were performed using the Biomek NXP liquid handler (Beckman Coulter). For data analysis, luminescence from the negative control well was averaged for each cell line at each time point, and results were normalized accordingly. ‘Non-lethal’ compounds were defined as drugs that consistently led to <30% inhibition for both diploid and aneuploid cell lines at all time points. ‘Lethal’ compounds were defined as drugs that consistently led to >30% inhibition after 48 h exposure and >60% inhibition after 72 h exposure. ‘Hit’ compounds were defined as drugs that consistently led to >20% difference in the response of diploid versus aneuploid cells, so that aneuploid cells responded more strongly to these drugs at least at one time point. Two screens were conducted for each pair of cell lines (CSES10 versus CSES22, HUES9 versus HUES7), and the combined results were then used for compound categorization. Z′ factors were calculated according to the formula: . Information on the compounds was obtained from the NCI/DTP website, according to their NSC ID numbers. Three ‘hit’ compounds were selected for confirmation: etoposide, cytarabine hydrochloride and gemcitabine hydrochloride (Sigma-Aldrich). Triplicates of all four cell lines were manually screened against multiple concentrations of these drugs for a 48-h exposure duration. Statistics Unsupervised hierarchical clustering and volcano plots were performed and visualized with Partek Genomics Suite version 6.3 (Partek). One-way ANOVA was performed with Partek Genomics Suite, with the following thresholds: fold-change >2, FDR-corrected P -value <0.05. Principal component analysis was performed and visualized using the R programming language and environment for statistical computing ( http://www.r-project.org/ ). For DAVID functional annotation analysis, significance was determined as P <0.05 after applying Benjamini–Hochberg correction. For PRIMA promoter enrichment analysis, significance was determined as P <1.0E-4 (the default value). Significance of overlap between gene lists was determined by Pearson’s χ 2 goodness-of-fit test. In the proliferation, viability and FACS experiments, and in the teratomas’ weight comparison, the significance of the differences between diploid and T12-hPSCs was determined by one-tailed Student’s t -test. The significance of the difference in recovery rate of pluripotent-like cells between diploid and T12-hPSCs was determined by one-tailed Fisher’s exact test. Accession codes: Microarray data have been deposited in Gene Expression Omnibus under the accession number GSE51455 . How to cite this article : Ben-David, U. et al. Aneuploidy induces profound changes in gene expression, proliferation and tumorigenicity of human pluripotent stem cells. Nat. Commun. 5:4825 doi: 10.1038/ncomms5825 (2014).